High pressure partially ionic phase of water ice Water ice dissociates into a superionic solid at high temperature (>2,000 K) and pressure, where oxygen forms the lattice, but hydrogen diffuses completely. At low temperature, however, the dissociation into an ionic ice of hydronium (H 3 O) + hydroxide (OH) − is not expected because of the extremely high energy cost ( ∼ 1.5 eV) of proton transfer between H 2 O molecules. Here we show the pressure-induced formation of a partially ionic phase (monoclinic P 2 1 structure) consisting of coupled alternate layers of (OH) δ− and (H 3 O) δ+ (δ=0.62) in water ice predicted by particle-swarm optimization structural search at zero temperature and pressures of >14 Mbar. The occurrence of this ionic phase follows the break-up of the typical O–H covalently bonded tetrahedrons in the hydrogen symmetric atomic phases and is originated from the volume reduction favourable for a denser structure packing. Water ice belongs to an important group of archetypal binary compounds with a large abundance in the interiors of giant planets [1] , [2] . The cores of Uranus, Neptune, Saturn and Jupiter are assumed to contain largely of water ice at pressures up to 40 Mbar (ref. 1 ). Thus, the ultra-high pressure studies on the structure properties of ice is of crucial importance for the understanding of the physics and chemistry of planetary interiors and even origin of their magnetic field distribution [3] , [4] , [5] . However, the conditions as occurring in the cores of giant plants are not directly experimentally accessible, as an alternative ab initio simulations are able to explore states of matters under such extreme conditions. Ice has a very rich phase diagram. Till now, at least 15 solid phases have been identified experimentally [6] , [7] and 4 other high-pressure phases were theoretically predicted [8] , [9] . Experimentally, all crystalline phases except ice X are found to consist of water molecules (each has two O–H covalent bonds) connected by hydrogen bonds. At low temperature and pressures above 70 GPa, ice dissociates and stabilizes at phase X, an atomic crystal having the symmetrical hydrogen bonds with each O atom covalently bonded to four H atoms. No higher-pressure phases beyond ice X have been experimentally verified up to the highest pressure 2.1 Mbar investigated so far. Theoretically, first-principles simulations established that an orthorhombic Pbcm phase surpasses ice X at ∼ 3 Mbar (ref. 8 ) and is energetically more stable than the earlier anti-fluorite structure [10] . Very recently, three 0 K crystalline Pbca, Pnma and Cmcm structures stable above 7.6 Mbar are proposed by a simulated annealing method [9] . These later theoretical atomic structures of post-ice X share the similarity with ice X, possessing fourfold O–H covalent bonds. Of particular interest is the recent finding of superionic ice at high temperatures (>2,000 K) and high pressures 5,6 , where oxygen remains fixed at the lattice, but hydrogen atoms diffuse completely. This superionicity is a clear temperature-driven phenomenon, allowing the break-up of the O–H covalent bond. At low temperature, however, the hydrogen atoms remain covalently bonded with oxygen where hydrogen transfer between two H 2 O molecules is energetically very unfavourable with a large energy cost (for example, 1.5 eV in solid [11] ). Therefore, the finding of ionic forms in ice at low temperature is scarce. To date, the dissociation of a H 2 O molecule in liquid water into (OH) − and (H 3 O) + at ambient pressure, and its high pressure enhancement have been reported [12] , [13] , [14] , but it is, in general, rare, short-lived and dynamically controlled. Here we report the direct prediction of formation of a partially ionic phase in water ice consisting of coupled alternate layers of (OH) δ− and (H 3 O) δ+ (δ=0.62) through our recently developed particle swarm optimization (PSO) algorithm for crystal structure prediction [15] at zero temperature and pressures (>14 Mbar). We also predict that a tetrahedrally O–H bonded covalent ice (tetragonal I- 42 d structure) containing highly distorted O–H tetrahedrons surpasses other known ice phases above 8.1 Mbar, bridging the hydrogen symmetric atomic phases with the ionic phase. Crystal structures Our structure searches through CALYPSO (Crystal structure AnaLYsis by Particle Swarm Optimization) code [15] with system sizes up to eight H 2 O formula units (f.u.) per simulation cell through both global and local PSO schemes, were performed at 2, 5, 7, 10, 15 and 20 Mbar. The experimental ice X and earlier theoretical Pbcm , Pbca , Pnma and Cmcm structures were all successfully reproduced in certain pressure ranges through both PSO techniques, validating our methodology in application to dense ice. We newly predicted two energetically favourable structures: a tetragonal I- 42 d (16 f.u. or cell, Fig. 1a ; Supplementary Table S1 ) and a monoclinic P 2 1 (4 f.u. per cell, Fig. 1b; Supplementary Table S1 ). I- 42 d structure containing two interpenetrating hydrogen-bonded networks, which can only be found by the more efficient local PSO scheme, shares the bonding similarity to earlier Pbcm and Pbca structures with each O atom bonded with four H atoms, but achieves denser structure packing with stronger bond–angle distortions in the tetrahedrons (for example, at 10 Mbar the H–O–H bond–angle distribution in I- 42 d structure extends from 92 to 127° instead of from 86 to 127° in Pbca ). Intriguingly, in P 2 1 structure, the structural feature of O–H tetrahedrons is no longer preserved. Instead, we find the surprising occurrence of alternate layers of OH and H 3 O units ( Fig. 1b ), implying the ionic nature of this solid. It should be noted that after the submission of this work, we became aware of an unpublished paper (arXiv:1106.1941v1) by McMahon, reporting the similar P 2 1 structure and a different lower pressure structure Pmc 2 1 , which, however, is energetically less favourable than our I -42 d structure. 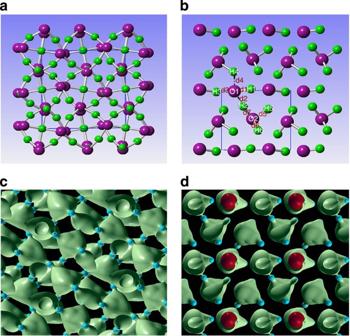Figure 1: Crystal structures and ELF Isosurfaces. (a) Crystal structure ofI-42dviewed along thecaxis. (b) Crystal structure ofP21viewed alongaaxis. The large spheres represent the oxygen atoms whereas the small ones are for hydrogen atoms. The atoms and O–H distances are labelled in accordance with the notation inTable 1. (c) Isosurface of ELF forI-42dstructures at 14 Mbar with the ELF value of 0.75. (d) Isosurface of ELF forP21structures at 14 Mbar with the ELF value of 0.75. Figure 1: Crystal structures and ELF Isosurfaces. ( a ) Crystal structure of I- 42 d viewed along the c axis. ( b ) Crystal structure of P 2 1 viewed along a axis. The large spheres represent the oxygen atoms whereas the small ones are for hydrogen atoms. The atoms and O–H distances are labelled in accordance with the notation in Table 1 . ( c ) Isosurface of ELF for I- 42 d structures at 14 Mbar with the ELF value of 0.75. ( d ) Isosurface of ELF for P 2 1 structures at 14 Mbar with the ELF value of 0.75. 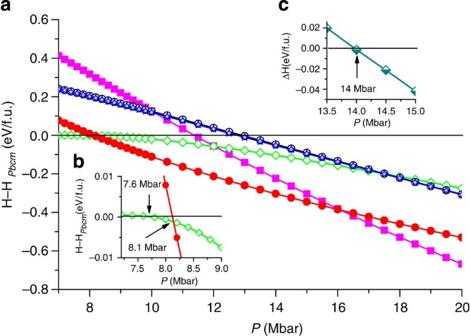Figure 2: Energetic stability as a function of pressure. (a) Calculated enthalpies (H) per H2O unit as a function of pressure (P) for various structures with respect toPbcmstructure. The green, blue and black lines indicate the enthalpies forPbca,PnmaandCmcm, respectively. The enthalpies ofI-42dandP21structures are marked by the red and pink lines, respectively. (b) The enthalpies (7.2–9 Mbar) ofPbcaandI-42dstructures with respect toPbcmin more details. (c) The enthalpies ofP21structure with respect toI-42dstructure with ZPE included. Full size image Structural stability The enthalpies of the predicted stable phases, calculated at higher levels of accuracy, are plotted as a function of pressure in Figure 2a . It is seen that ice transforms from Pbcm to Pbca at 7.6 Mbar ( Fig. 2b ), in excellent agreement with earlier theoretical calculations [9] . The Pbca structure is stable at 7.6–8.1 Mbar, above which the I- 42 d structure takes over and exists in a large pressure range till 16 Mbar, where P 2 1 structure becomes most energetically favourable up to 20 Mbar, the highest pressure studied. Note that the zero-point energy (ZPE) is not included in the enthalpy calculations, which can be very large owing to the small atomic masses of H and O atoms. Indeed, our estimated ZPEs for Pbca and I- 42 d structures at 10 Mbar by a quasi-harmonic model [16] have large values of 1.105 eV f.u. −1 and 1.110 eV f.u. −1 , respectively. However, their difference is very small, giving a negligible modification on the transition pressure of Pbca → I- 42 d . Interestingly, P 2 1 structure has a much smaller ZPE (1.148 eV f.u. −1 ) than that of I- 42 d structure (1.229 eV f.u. −1 ) at 14 Mbar, lowering the I- 42 d → P 2 1 transition pressure from 16 to 14 Mbar ( Fig. 2c .) The physical origin of smaller ZPE in P 2 1 structure is largely related to the gross weaker O–H covalent bonding as evidenced by the averaged larger O–H bond lengths (for example, at 14 Mbar, the average O–H bond length is 1.03 Å for P 2 1 structure to compare with 0.97 Å for I- 42 d structure). It should be noted that both I- 42 d and P 2 1 structures are dynamically stable in their stability fields ( Supplementary Fig. S1 ). Figure 2: Energetic stability as a function of pressure. ( a ) Calculated enthalpies (H) per H 2 O unit as a function of pressure (P) for various structures with respect to Pbcm structure. The green, blue and black lines indicate the enthalpies for Pbca , Pnma and Cmcm , respectively. The enthalpies of I -42 d and P 2 1 structures are marked by the red and pink lines, respectively. ( b ) The enthalpies (7.2–9 Mbar) of Pbca and I- 42 d structures with respect to Pbcm in more details. ( c ) The enthalpies of P 2 1 structure with respect to I- 42 d structure with ZPE included. Full size image Chemical bondings The unexpected formation of OH and H 3 O units invites us to perform a thorough analysis on the chemical bondings of P 2 1 structure. We first calculated the electron localization functions (ELF), known to be an informative tool to distinguish different bonding interactions in solid [17] . The isosurface plots at ELF=0.75 (a typical good number for characterization of covalent bondings) [17] clearly illustrate the covalent bonding nature of the I- 42 d structure ( Fig. 1c ) and confirm the formation of OH and H 3 O units in P 2 1 structure ( Fig. 1d ; Supplementary Fig. S2 ). However, we also noticed a small charge distribution localized in between OH and H 3 O, an indicative of their covalent interaction. We subsequently performed a topological analysis of the static electron density through Bader's quantum theory of atoms-in-molecules [18] , which has been successfully applied to the determination of bonding interactions through the values of the density and its Laplacian at bond critical points. The calculated data are summarized in Table 1 . Again, the analysis gives strong evidence on the formation of OH and H 3 O units as indicted by the very negative values of the Laplacian of charge density at the critical points. In agreement with above ELF results, our calculation also supports the covalent interaction (though relatively weak) between OH and H 3 O layers as seen from the noticeable negative Laplacian value ( Table 1 ) between O1 and H2/H3/H4 (d2, d3 and d4 in Fig. 1b ). This interaction is understandable because P 2 1 structure is a highly packed structure at such an extreme pressure of 14 Mbar (at higher pressure 20 Mbar, this interaction becomes even stronger as shown in Table 1 ). The two identities are too close to not be covalently interacted. However, this covalent coupling is, in fact, not intrinsic as we find the interaction decreases significantly with lowering pressure to 7 Mbar ( Table 1 ), whereas the extraordinarily strong O–H bondings within OH and H 3 O units remain nearly unaltered, and at an extreme case by extrapolation to about 2 Mbar, no interaction was found at all. To support our argument, we have theoretically compressed the perfect ionic NH 4 + NH 2 − solid derived from NH 3 (ref. 19 ) and found a similar covalent interaction of NH 4 + and NH 2 − at a pressure 7 Mbar. On the basis of Bader theory [18] , the approximate charge values of oxygen and hydrogen ions of P 2 1 structure are calculated at 14 Mbar as listed in Table 2 . We found different charges for inequivalent oxygen and hydrogen ions as determined by their distinct chemical environments. It is seen that the charge transfer from H 3 O to OH is about 0.62 e at 14 Mbar, illustrating the ionic nature of P 2 1 structure with a notation of (OH) δ − (H 3 O) δ + ( δ =0.62). Table 1 Bond critical point data of P 2 1 structure. Full size table Table 2 Bader charges of oxygen and hydrogen ions in P 2 1 structure. Full size table Electronic structures The calculated electronic band structures ( Supplementary Fig. S3 ) for I- 42 d and P 2 1 structures reveal that the two phases are both insulators with large band gaps (>5.0 eV at 14 Mbar for P 2 1 structure), which show weak dependence on pressure (for example, at a rate of −0.135 eV Mbar −1 for P 2 1 structure). Considering also that density-functional calculations usually underestimate the band gaps, we expect that the low-temperature metallization of ice is only possible at pressures much higher than 20 Mbar. Our results are in apparently contrast to the earlier proposal on the metallicity of ice at 15.5 Mbar (ref. 9 ). Above 3 Mbar, ice X transforms into Pbcm , Pbca , and I- 42 d structures, which all contain distorted O–H tetrahedrons (oxygen is in the centre, whereas hydrogen atoms occupy the tetrahedral sites) where hydrogen atoms are squeezed out of midpoint between oxygen atoms. These transformations follow the continuous distortion of O–H tetrahedrons with severer H deviations (for example, the enlarged H–O–H angles), but the tetrahedrons remain. Eventually, at the formation of P 2 1 structure, the typical O–H tetrahedrons in the atomic phases collapse completely ( Fig. 1a,b ). We contribute the phase transformations to the needs for denser structure packing driven by pressure ( Supplementary Fig. S4 ). Our calculations show that the sphere packing efficiency at 14 Mbar increases continuously in the order of 25.5%→29.4%→32.1%→33.93%→35.44% for ice X, Pbcm , Pbca , I- 42 d , and P 2 1 structure, respectively. As is known that Gibbs free energy reduces to H=U+PV at 0 K, where U, P and V are the static energy, pressure and volume per formula unit, respectively. The high pressure competition between U and PV dominate the phase transitions. Although, the first order transitions of Pbca → I- 42 d → P 2 1 have rather small 1.8% and 1.9% volume drops, respectively, these volume reductions are critical to initiate the phase transitions. It is calculated that although P 2 1 structure is 0.59 eV per H 2 O unit higher in U than I- 42 d structure at 17 Mbar, its PV term is 0.62 eV lower owing to the volume reduction associated with a higher packing efficiency. The pressure-induced formation of ionic solid on molecular systems has been predicted theoretically for NH 3 (ref. 19 ), H 2 S [20] and NH 3 ·H 2 O [21] and observed experimentally for N 2 O [22] . The dissociation of H 2 S into SH − and SH 3 + is short lived and dynamically controlled [20] , similar to that in liquid water [12] , [13] , [14] , [23] . The stabilization of NO 3 − NO + solid compressed from N 2 O violates the conservation of chemical composition and there temperature has had a significant role on its formation [22] . Our finding in some ways resembles with the ionic mechanism of NH 3 (ref. 19 ) and NH 3 ·H 2 O [21] solids. What makes the ionicity in H 2 O unique is the existence of covalent coupling between OH and H 3 O, leading to a partial ionicity. Notably, the ionic pressure ( ∼ 14 Mbar) in H 2 O is considerably higher than ∼ 1 Mbar in NH 3 (ref. 19 ) and 0.05 Mbar in NH 3 ·H 2 O [21] . The physical origin behind this high ionic pressure is stemmed from the much larger energy barrier ( ∼ 1.5 eV [11] ) of proton transfer between two H 2 O molecules. The current findings of high-pressure phases of I- 42 d and P 2 1 structures have enriched the chemical bondings of ice, and substantially extended the low-temperature phase diagram of ice to the pressure ranges of 8.1–20 Mbar, relevant to the interiors of giant planets. Our results may be useful as the initial low-temperature structures to build up the constituent model for planetary interiors at high temperature. Our prediction of partially ionic ice is unusual in view of the existence of large energy barriers of hydrogen transfer between two H 2 O molecules, but highlights the critical role pressure had in overcoming the energy barriers. Energetically, the tuning effect of PV term with respect to static energy U is substantial in light of volume reduction preferable for denser structural packing. In the same manner, ionicity might be expected in other molecular systems (for example, CO 2 , NO 2 and so on), not at low but extreme pressures. Crystal structure prediction Our structure search simulations are performed through the CALYPSO method [24] as implemented in CALYPSO code [15] , which is specially designed for global structural minimization unbiased by any known structural information. Our approach is based on a global minimization of free-energy surfaces merging ab initio total-energy calculations via PSO technique [24] . Our CALYPSO method has been benchmarked on various known systems [24] with various chemical bondings and had several successful prediction of high-pressure structures of Li, Mg and Bi 2 Te 3 (refs 25 , 26 , 27 ), among which the insulating Aba 2–40 (or oC40) structure of Li and the two low-pressure monoclinic structures of Bi 2 Te 3 have been confirmed by independent experiments [27] , [28] . We have adopted a local PSO scheme, which was designed to avoid the premature structure convergence by maintaining multiple attractors and to allow the exploration of larger space of free-energy surfaces. Therefore, the local PSO is computationally more demanding, but more effective than global PSO technique, particularly when simulation sizes are larger than 24–30 atoms per cell where the free-energy landscape is more complex. Detailed description of the method and predictions can be found in the Supplementary Methods . Total energy calculations Total energy calculations were performed in the framework of density functional theory within the Perdew–Burke–Ernzerhof [29] parameterization of generalized gradient approximation [30] as implemented in the VASP (Vienna Ab Initio simulation package) code [31] . The projector-augmented wave (PAW) method [32] , [33] was adopted with the PAW potentials taken from the VASP library where 1 s 1 and 2 s 2 2 p 4 are treated as valence electrons for H and O atoms, respectively. The validity of the used PAW potential at currently studied pressures (<20 Mbar) has earlier been carefully checked by comparing with the full-potential all-electron calculations through Exciting code [9] . The use of the plane-wave kinetic energy cutoff of 1,200 eV and dense k-point sampling [34] , adopted here, were shown to give excellent convergence of total energies. How to cite this article: Wang, Y. et al . High pressure partially ionic phase of water ice. Nat. Commun. 2:563 doi: 10.1038/ncomms1566 (2011).